X-ray holography with a customizable reference In X-ray Fourier-transform holography, images are formed by exploiting the interference pattern between the X-rays scattered from the sample and a known reference wave. To date, this technique has only been possible with a limited set of special reference waves. We demonstrate X-ray Fourier-transform holography with an almost unrestricted choice for the reference wave, permitting experimental geometries to be designed according to the needs of each experiment and opening up new avenues to optimize signal-to-noise and resolution. The optimization of holographic references can aid the development of holographic techniques to meet the demands of resolution and fidelity required for single-shot imaging applications with X-ray lasers. X-ray Fourier-transform holography (FTH) [1] , [2] , [3] is a robust coherent imaging technique that has found wide-ranging applications to biology [2] and material science [3] . The technique is particularly suited to imaging magnetic domains and other magnetic samples because holograms generated with circularly polarized X-rays can be used to separate charge scattering from magnetic scattering [3] , [4] , [5] . X-ray holography has developed into a powerful single measurement technique [1] , [6] and has promising applications using X-ray lasers to study structures of radiation-sensitive samples and the structural changes of transient phenomena [6] , [7] , [8] . The definitive feature of holography is the use of a reference wave to facilitate a simple, direct and robust image-reconstruction procedure. However, to date the choice of reference wave in FTH has been restricted to those few cases for which the analytic image-reconstruction procedure is known. This in turn places restrictions on the sample-reference geometry and experimental design. Here we introduce a general image-reconstruction procedure for FTH data that places minimal restrictions on the reference, enabling a much greater flexibility for the design of X-ray holographic experiments. The simplest choice of FTH reference is a pinhole in the sample plane, and it was this reference that was used in the first demonstrations of X-ray holography [3] , [9] . It is a convenient reference because the hologram is obtained by a single Fourier transform of the measured data. The resolution of the hologram is determined by the diameter of the pinhole, which has the unfortunate consequence of coupling flux and resolution. To improve resolution while maintaining flux, multiple pinholes can be used [10] . However, adjacent pinholes must be sufficiently separated to produce non-overlapping holograms and consequently the field-of-view is used inefficiently. Alternatively, flux and resolution can be decoupled by using extended references [1] , [11] , [12] , [13] . The image-reconstruction procedure for extended references involves the application of linear operators, such as convolution [1] , linear filters [11] , [12] or propagation [13] . However, there are only a handful of special cases for which these reconstruction procedures are known. Notwithstanding the specificity of each approach, the aforementioned methods still leave something to be desired as Fresnel-zone plate references have missing information at low frequencies [13] and sharp corner references improve resolution only along a few specific directions [14] . A further limitation is that missing data have a significant impact on the results of existing FTH methods. High-intensity X-rays in the forward direction are usually blocked by a beam stop or allowed to pass by gaps in modular detectors, creating regions of missing data that are not accounted for in many existing reconstruction procedures. There are in fact many more possible reference waves for holographic experiments than have been demonstrated in X-ray holography to date [15] . It is possible to recover images from a large class of reference waves by formulating the holographic image reconstruction within a general framework that leads to a system of linear equations. The linear equations are efficiently and robustly solved by the iterative linear reconstruction using Fourier transforms method (ILRUFT) [16] , which is based on the least-squares conjugate-gradient method [17] . This approach has been successfully applied in the context of electron coherent diffractive imaging (CDI) [18] and electron ptychography [19] . Here we develop ILRUFT into a generalized X-ray holography technique and provide a proof-of-principle demonstration that highlights its potential for single-shot femtosecond imaging with X-ray lasers using arbitrary illumination. Our implementation of ILRUFT for X-ray holography allows for the handling of missing data, a feature that is particularly useful for single-shot applications with X-ray lasers, where missing data regions are typically large. ILRUFT for X-ray holography Although the ILRUFT method has been described in detail elsewhere [16] , it will be valuable here to briefly summarize the central ideas before discussing the specific developments required for X-ray holography. The X-ray wave at the exit surface plane of the object can be decomposed into the sum of scattered waves from the object and the reference, as follows If the diffraction pattern is composed of multiple exposures then represents the average of all the reference waves, as discussed further in Methods. By taking an inverse Fourier transform of the measured diffraction data (assuming there are no missing data), the autocorrelation of the exit wave A data is obtained, and may be expressed as where A ref and A obj are the autocorrelation functions of the reference and object waves, respectively, and C ref,obj are the cross-correlations between the reference and the object waves. As explained in detail in ref. 15 , when the object is finite, there are large regions of the autocorrelation function where A obj =0, and in this region equation (2) can be reformulated as The matrix consists of values of . Since the reference wave is assumed to be known a priori and the cross-correlations can be reliably extracted from the measured data, both A ref and are known and we can solve equation (3) as a system of linear equations for the unknown scattered wave, . Furthermore, an efficient solution to the set of equations can be obtained using the conjugate-gradient least-squares algorithm within the ILRUFT framework, where the action of the matrix and its transpose on a vector can be formulated efficiently with Fourier transforms, and need never be constructed explicitly. When the diffraction pattern contains regions of missing data, say, for example, through the use of a beam stop, it is necessary to account for the way in which missing data affect the autocorrelation functions and consequently the set of linear equations need to be modified. We define a binary mask that takes the value one on pixels where data were measured and zero otherwise. The linverse Fourier transform of the mask is defined by (where is the Fourier-transform operator). When there are missing data, ILRUFT is applied by making the following substitutions and where ⊗ represents a convolution. As the function P has an extended width, the nonlinear term P ⊗ A obj is no longer confined to the central region of the exit-wave autocorrelation function but expands to contaminate regions where the linear equations would have otherwise been in isolation. We treat this contamination as an additional source of error. If the missing data region is not too extensive, a significant fraction of the linear equation region is not greatly affected by the spreading of the nonlinear information. This and other sources of error (for example, measurement noise) are accommodated through regularization via iteration number in the ILRUFT algorithm. As with CDI techniques, if the extent of the missing data exceeds the width of a speckle (a diffraction fringe with a minimum width), then the reconstructed image will not contain low-frequency information that can affect contrast [20] . The amount of unmeasured object information can be characterized by a modal analysis [21] . These considerations and their impact on our generalized holographic approach and the accompanying experimental results will be discussed further below. The use of a priori knowledge about the scattered wave is a common practice in conventional X-ray CDI, and may also be included in the generalized scheme presented here. Reality and positivity are two object constraints that are commonly used. In the present case we can restrict to be a real function by setting its imaginary component to zero in equation (3). Positivity cannot be incorporated directly into the conjugate-gradient least square iterations because it impedes convergence and alternative non-negative least square solvers that have been reported in the literature [22] , [23] do not lend themselves to an efficient FFT-based implementation such as ILRUFT. Nevertheless, the conjugate-gradient iterations can be periodically terminated to enforce positivity. It was found that after the first application of the positivity constraint the reconstructed image was already of a sufficiently high quality, and further conjugate-gradient iterations were not necessary. Experiment The references for our experiment were chosen to be significantly different to each other as well as those currently used in FTH. We begin by considering two cases, one with a partial circle and another with a ‘cartoon-cloud’ reference ( Fig. 1a,b , respectively). The continuous curved features of these references differ markedly from the straight-edged features of corner holography and references constructed of pinholes. The continuous enclosure of an object by the reference structure deviates from the usual requirement of a reference that is isolated and contained to a small local region. This indicates how flexibly we can make use of the field-of-view. 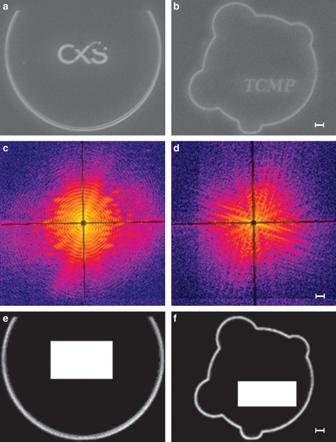Figure 1: Samples and diffraction patterns. The SEM images of the samples are shown ina,b. The diffraction patterns of the two samples are shown inc,dwith the central shaded areas indicating regions that have been set to zero for the reconstructions. The reference functions estimated from the SEM images are shown ine,falong with the assumed object areas indicated by the white rectangles. The scale bars inb,frepresent 500 nm and the scale bar indrepresents 0.1 μm−1. Imagesa,b,eandfare on the same scale. Imagescanddare on the same scale. Figure 1: Samples and diffraction patterns. The SEM images of the samples are shown in a , b . The diffraction patterns of the two samples are shown in c , d with the central shaded areas indicating regions that have been set to zero for the reconstructions. The reference functions estimated from the SEM images are shown in e , f along with the assumed object areas indicated by the white rectangles. The scale bars in b , f represent 500 nm and the scale bar in d represents 0.1 μm −1 . Images a , b , e and f are on the same scale. Images c and d are on the same scale. Full size image For the general holographic method here, it is necessary that the spatial separation between some point on the reference and the object is at least of one object width in order to produce a sufficient number of linearly independent equations [15] . These requirements do not exclude references that approach or even overlap the sample, although knowledge of the reference in the overlap region will not contribute the coefficients of in equation (3) and plays no part in the reconstruction procedure. The experiment was performed at FERMI [24] , [25] , [26] , a seeded soft X-ray free-electron laser. It is a highly suitable source for coherent X-ray imaging because of its high brightness and excellent coherence properties [8] . Our test objects were fabricated on Si 3 N 4 windows using a focused ion beam (see Methods), similar to other CDI experiments [8] , [27] . Scanning-electron microscope (SEM) images of the two samples are shown in Fig. 1a,b . Diffraction patterns recorded from 50 and 100 exposures for the Coherent X-ray science (CXS) and Theoretical condensed matter physics (TCMP) samples are shown in Fig. 1c,d , respectively. Data contained large crossed streaks that arise from X-ray scattering from the edges of the Si 3 N 4 window. These streaks needed to be masked before reconstruction and are indicated by the shaded central regions. While this removes a sizable fraction of data, it is comparable to the amount of missing data present when using modular detectors in XFEL experiments [28] . A missing mode analysis [21] identified one weakly constrained mode for the ‘CXS’ object, and none for ‘TCMP’, indicating that the likelihood of reconstruction ambiguities due to the missing data are low (see Methods). The test objects consisted of two distinct objects on each window, of which one was designated as the reference. An estimate of the reference for each case, shown in Fig. 1e,f , was made from the SEM image of the sample (see Methods). We assume that the average illumination over multiple exposures is uniform, ignoring the impact of the non-uniform illumination profile as discussed further in the Methods section. With ILRUFT the use of a tight support is not necessary. The size of the assumed object areas were overestimated and are shown in Fig. 1e,f by the white rectangles. The analysis of the exit-wave autocorrelation used to set up the ILRUFT reconstruction is discussed further below in Methods. It is crucial to have an accurate centring of the diffraction pattern and an accurate reference wave intensity to produce the highest-quality image. These parameters were refined by searching for values that minimized the residual error [29] . To further improve the robustness of the reconstruction, reality and positivity constraints were applied, as described above. Applying the generalized holographic reconstruction procedure to the diffraction data produced the reconstructions for the test objects as shown in Fig. 2a,b . In both cases a clear image is recovered for each example test object. 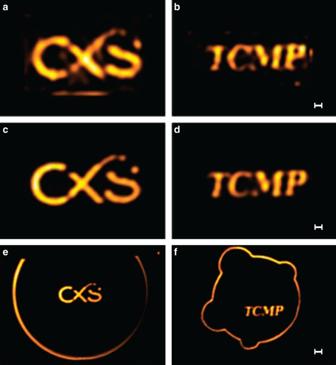Figure 2: Reconstructed images. The object intensities reconstructed by ILRUFT are shown ina,band those reconstructed by RAAR are shown inc,d. The full exit surface wave intensity reconstructed by RAAR is shown ine,f. The scale bars shown inb,drepresent 200 nm and the scale bar infrepresents 500 nm. Imagesa–dare on the same scale. Imageseandfare on the same scale. Figure 2: Reconstructed images. The object intensities reconstructed by ILRUFT are shown in a , b and those reconstructed by RAAR are shown in c , d . The full exit surface wave intensity reconstructed by RAAR is shown in e , f . The scale bars shown in b , d represent 200 nm and the scale bar in f represents 500 nm. Images a – d are on the same scale. Images e and f are on the same scale. Full size image We compared the ILRUFT holographic reconstruction with a non-holographic nonlinear iterative CDI reconstruction. Successful reconstructions were obtained using the relaxed-alternating-averaged reflection (RAAR) algorithm [30] , shown in Fig. 2c,d , which are very similar to the ILRUFT reconstructions. The estimated reference was provided as input, and the assumed object area was set to random values. The RAAR reconstruction used no a priori knowledge of the test object other than the reference wave. Seeding the RAAR without the SEM-derived reference wave resulted in failed reconstructions or slow convergence. The best reconstructions were obtained when RAAR was able to refine both reference and object and the initial support was allowed to vary using the shrinkwrap algorithm [31] . The refined exit surface waves produced by RAAR are shown in Fig. 2e,f . Our general reconstruction method can be used with all of the references from existing FTH techniques. As an example we have performed a reconstruction with a uniformly redundant array (URA) reference, similar to that used by Marchesini et al. [1] The measured diffraction pattern is shown in Fig. 3a and the SEM image of the sample is shown in Fig. 3b . There are in fact two URA structures, in addition to the ‘CFEL’ sample. As a single exposure was used to record the diffraction data, the intensity of the illumination was not uniform across the two URAs because of the beam profile, and the best results were obtained by selecting the brightest URA as the reference. The estimated reference and assumed object areas for the ILRUFT reconstruction are shown in Fig. 3c . The ILRUFT result, shown in Fig. 3d , is very similar to the RAAR reconstruction, shown in Fig. 3e . Owing to the missing data, reconstructing the object by convolution, as shown in ref. 1 , is exceedingly challenging. To reduce the artifacts in the autocorrelation plane, a high-pass filter with a Guassian profile (see Methods) was applied to the diffraction pattern before performing the convolution. Our best result, shown in Fig. 3f , does not produce a clear image of either the ‘CFEL’ object or the URA object. Curiously, the centre of the convolved autocorrelation function, located in the top left corner of Fig. 3f , reproduces an image of the URA reference itself. This is the contribution from the A ref term in equation (2). The ILRUFT reconstruction demonstrates a distinct advantage for working with missing data over a reconstruction by convolution. 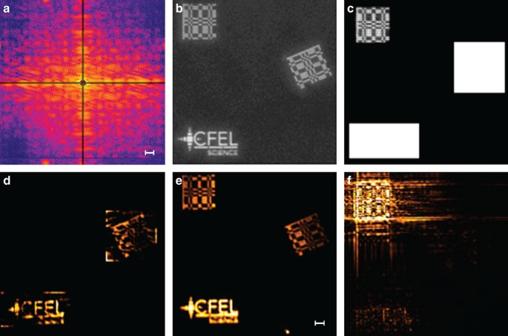Figure 3: URA reconstructions. The diffraction pattern of the URA reference case is shown ina, and the SEM image of the sample is shown inb. The estimated reference function is shown inc, and the areas assumed to contain the objects are indicated by the white rectangles. The intensity of the ILRUFT reconstruction is shown ind, the intensity of the averaged RAAR reconstruction is shown ineand the reconstruction by convolution is shown inf. Note thatfhas been cropped so that the centre is located in the top left corner, so that only the most relevant part for comparison to the other reconstructions is shown. The scale bar inarepresents 0.1 μm−1. The scale bar inerepresents 500 nm and imagesb–fare on the same scale. Figure 3: URA reconstructions. The diffraction pattern of the URA reference case is shown in a , and the SEM image of the sample is shown in b . The estimated reference function is shown in c , and the areas assumed to contain the objects are indicated by the white rectangles. The intensity of the ILRUFT reconstruction is shown in d , the intensity of the averaged RAAR reconstruction is shown in e and the reconstruction by convolution is shown in f . Note that f has been cropped so that the centre is located in the top left corner, so that only the most relevant part for comparison to the other reconstructions is shown. The scale bar in a represents 0.1 μm −1 . The scale bar in e represents 500 nm and images b – f are on the same scale. Full size image Each pixel in the images is 58 nm in width, and features across three pixels are clearly seen in all images, indicating a half-period resolution of ~170 nm. To confirm this estimate, the reconstruction was used to estimate the average diffraction intensity as a function of resolution shell and compared with the measured data in Fig. 4 . The reconstructed diffraction intensity of both RAAR and ILRUFT reconstructions of the TCMP and CXS objects matches the measured intensity well to a half-period resolution of 170 nm, at which point the reconstructed intensity drops, indicating higher-resolution information was not recovered. The resolution for the RAAR reconstruction was confirmed by constructing a phase retrieval transfer function [32] from 80 trials with random initial objects. The phase retrieval transfer function (not shown) fell to a value of 0.5 at 150-nm half-period resolution. The RAAR reconstruction intensity with the URA reference also extends to ~170 nm, but notably the ILRUFT reconstruction contains an intensity similar to the measured diffraction out to the edge of the detector. 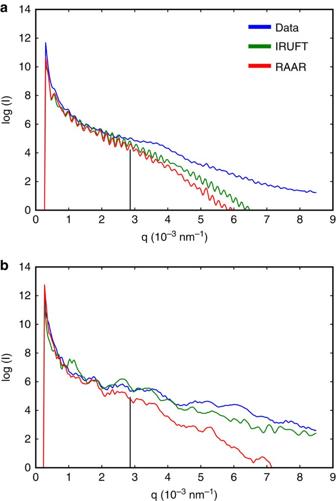Figure 4: Comparing measured and reconstructed diffraction intensities. The average intensity per detector pixel as a function of scattering vector q for the TCMP object (a) and the URA reference (b). The measured diffraction patterns are compared with the diffraction patterns modelled from the ILRUFT and RAAR reconstructions. The vertical black line indicates a full-period resolution of 350 nm (175 nm half-period resolution). The plot for the CXS object is very similar to that for the TCMP object and has been omitted. Figure 4: Comparing measured and reconstructed diffraction intensities. The average intensity per detector pixel as a function of scattering vector q for the TCMP object ( a ) and the URA reference ( b ). The measured diffraction patterns are compared with the diffraction patterns modelled from the ILRUFT and RAAR reconstructions. The vertical black line indicates a full-period resolution of 350 nm (175 nm half-period resolution). The plot for the CXS object is very similar to that for the TCMP object and has been omitted. Full size image The reference structures refined during the RAAR reconstructions display low-frequency variations of contrast that are inconsistent with the assumed uniform contrast used as input for the ILRUFT reconstructions. These features in the RAAR reconstruction may be because of the beam profile or because of missing data effects, which could be exacerbated by the large support required to cover both object and reference. Providing the refined reference from the RAAR reconstruction as an input for a new ILRUFT reconstruction did not produce any significant improvement. There are one or two residual artifacts in the ILRUFT reconstructions, such as the horizontal line present below the ‘CXS’ ( Fig. 2a ), which indicate some remaining sources of error, such as measurement noise on the diffraction pattern, background scattering or inadequate reference characterization. Artifacts mostly occur at the edge or corners of the assumed object area as lines or dots not more than one or two pixels width. Hence, they are easily distinguished from the object’s structure and do not complicate the interpretation of the image. This is supported by the fact that enlarging the object area shifts the location of these artifacts in reconstructions (not shown). ILRUFT differs from other holography methods by using a reference wave defined by a pixelated image rather than by assuming an ideal analytic form. The reference wave is sensitive to sample composition and thickness, in addition to the shape. Although this suggests that ILRUFT requires a higher level of a priori knowledge than other holography methods, in practice a partial characterization of the reference wave does not cause ILRUFT to fail. The conjugate-gradient algorithm introduces elements of the solution with iteration in order of significance, so that the first iterations generally correspond to low-resolution reconstructions. An imprecise input reference wave introduces errors gradually with iteration number and still yields a resolution-limited image with a judicious termination of the algorithm. This is effectively the same regularization discussed previously to handle errors associated with measurement noise and missing data. In fact, if an accurate characterization of the reference wave is available, the ILRUFT method can be tailored to best use this information, potentially exceeding the performance of other methods. For example, the ILRUFT method could account for the aberrations of a Fresnel-zone plate reference [13] . It should be noted that other extended references, such as corner or URA references, impose requirements on the uniformity of reference composition and thickness. In this way, accurate reference fabrication is very important in holography generally. From the perspective of fabrication and a priori knowledge, a pinhole reference produces the simplest experiment because the hologram is readily interpreted as a blurred image of the object. However, with pinholes the trade-off between flux and resolution, as described above, is a significant disadvantage that motivates research into alternative holographic methods, where gains can be made by increasing experimental complexity. Similar to other holographic methods, the resolution of the ILRUFT reconstruction is limited by the highest spatial frequency of the reference wave scattering. Consequently, an extended reference used with the ILRUFT method would be limited by the gradient of the edge profile, similar to references with sharp corners [12] . The option is now available to design references that improve resolution in all directions simultaneously, avoiding the directional bias of corner references. Aside from the structured reference scatterers, as shown here, the reference could be provided by a structured beam like the convergent beams that have been used in Fresnel CDI (ref. 33 ). If the propagation between the sample and the detector is a Fresnel propagator, then no fabricated reference is required for ILRUFT [34] . In this case the form of the propagator provides the coefficients from which to construct . Sample preparation The reference and test objects were constructed using a focused ion beam to deposit platinum (~16%) and carbon (~84%) on a silicon nitride window. The Si 3 N 4 windows were 30-nm thick and the deposited structures were of the order of 10-nm thick. Experimental methods The pulses produced by FERMI had a wavelength of 32.5 nm and are estimated to be 100 fs in duration. The focal spot of the beam was ~15 × 30 μm 2 . After the gas attenuator the pulse energy was 10–15 μJ. The beam was attenuated by a further 1.25% by aluminium filters. Final measurements were made by integrating multiple pulses to the same window. The number of integrated pulses was chosen to be less than saturation and differed for each sample. The ‘CXS’ and ‘TCMP’ measurements were accumulated from 50 and 100 pulses, respectively. The URA measurement was obtained with a single shot, with reduced beam attenuation so that the total post-filter energy was 10 μJ. The diffraction patterns were acquired using a 32.5-nm multilayer mirror that reflects the scattered photons on a CCD detector (Princeton instrument MTE2048B, 13.5 μm pixel size) placed at ~55 mm from the interaction region. In order to avoid damage to the CCD camera from the direct FEL beam, the reflecting mirror has a hole of ~0.5 mm diameter. Using such experimental configuration, the maximum scattering angle is of about 14 deg with a missing data region of 0.4 deg. The maximum spatial frequency recorded by the detector was 2 π × 0.017 nm −1 . Reconstruction methods The reference was estimated from the SEM image by selecting the reference structure using a binary mask and applying a Gaussian noise filter. The filter was 2 pixels full-width at half-maximum. The reference size was scaled to match the size of features in the experimentally determined autocorrelation function (shown in Fig. 5a,b ). The normalization of the reference was determined by minimizing the residual error of the ILRUFT reconstruction [29] . 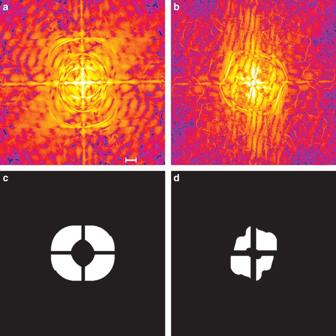Figure 5: Autocorrelation functions and linear equation regions. The amplitude of the autocorrelation functions generated from the inverse Fourier transform of the masked diffraction patterns (Fig. 1a,b) are shown ina,bon a log scale, cropped to show only the relevant regions for holographic ILRUFT analysis. The regions of linear equations assumed for the analysis are shown inc,d. The scale bar inarepresents 350 nm and all images are on the same scale. Figure 5: Autocorrelation functions and linear equation regions. The amplitude of the autocorrelation functions generated from the inverse Fourier transform of the masked diffraction patterns ( Fig. 1a,b ) are shown in a , b on a log scale, cropped to show only the relevant regions for holographic ILRUFT analysis. The regions of linear equations assumed for the analysis are shown in c , d . The scale bar in a represents 350 nm and all images are on the same scale. Full size image The linear equation regions, shown in Fig. 5c,d , were estimated by taking a cross-correlation of the reference domain and the assumed object area. Horizontal and vertical streaks in the horizontal and vertical directions are due to the spread of the nonlinear term, A obj , and were excluded from the linear equation region. The ILRUFT reconstruction was run for 15 iterations and took the order of minutes to compute. It was terminated when the ratio of the change in object intensity to the change in residual error began to sharply increase. At this point, further updates to the reconstructed objects did not improve the comparison with the experimental data and represented the addition of noisy information to the images. The RAAR reconstructions were run for 200 iterations, updating the support every 10 iterations. The RAAR feedback parameter ( β ) was 0.9. The shrinkwrap algorithm was implemented with a threshold of 15% of the maximum intensity of the object, after convolving with a Gaussian kernel. The half-width at half-maximum of the Gaussian kernel was reduced linearly from three pixels to one pixel during the reconstruction. Reality and positivity constraints were not applied. The convolution reconstruction with the URA reference was performed by convolving the experimentally determined exit-wave autocorrelation function with the estimated URA reference function ( Fig. 3b ). Before performing the convolution, a high-pass filter was applied to the autocorrelation function defined by , where r is a radial coordinate and σ was set to an eighth of the detector width. The filter reduced artifacts in the exit-wave autocorrelation function because of the missing data region, and the optimal width of the filter was chosen by visual inspection of the result. Data processing The mean offset value of the detector and any uniform background scattering was estimated from a 100 × 100 pixel corner region of the diffraction pattern and subtracted. A mask was created to remove the streaks from the window scattering and the central hole. The diffraction pattern was centred by computing the centre of mass of the diffraction pattern and later refined by minimizing the residual error in the ILRUFT reconstruction. Missing mode analysis A missing mode analysis [21] was performed using the object pixel basis to identify weakly constrained information about the object. Weakly constrained modes are functions that when added or subtracted from the reconstructed image have a minimal effect on the error metric minimized by the reconstruction algorithm. The reconstruction had one weakly constrained mode with a constraining power of 0.03; however, it had no apparent affect on the ILRUFT reconstruction after reality and positivity constraints were applied. The ‘CXS’ reconstruction with RAAR had no weakly constrained modes after the support was refined by shrinkwrap. The ‘TCMP’ reconstruction using ILRUFT had no weakly constrained modes and the minimum constraining power was 0.3. Integrating multiple exposures When the diffraction is accumulated from multiple exposures (indexed by i ) and the probe illumination fluctuates between exposures, the average cross-correlation between reference waves and object waves is This case can be accommodated by defining for the input to ILRUFT. The reconstructed object wave is then interpreted as the average of the object waves from each exposure. The second term affected by a variable probe is A ref , which is approximated by A source of pulse variability in our experiment was beam jitter in the sample plane and the average reference wave can correspond without the assumption of uniform reference contrast more closely than the reference wave for any individual exposure. Any errors that arise from these approximations are regularized by truncating the ILRUFT iteration as described above in the reconstruction methods. How to cite this article : Martin, A. V. et al. X-ray holography with a customizable reference. Nat. Commun. 5:4661 doi: 10.1038/ncomms5661 (2014).